Identification of active atomic defects in a monolayered tungsten disulphide nanoribbon Edge structures and atomic defects can significantly affect the physical and chemical properties of low-dimensional materials, such as nanoribbons, and therefore merit a thorough investigation at the atomic scale. Here, we successfully discriminate single atoms on a monolayered tungsten disulphide nanoribbon by means of time-resolved annular dark-field imaging and spatially resolved electron energy-loss spectroscopy. We unambiguously identify and successfully visualize in motion atomic defects, such as vacancies and edge atoms, using scanning transmission electron microscopy. We also report a direct observation of slip deformation in the nanoribbons and present evidence demonstrating that the deformation process involves the migration of vacancies and rearrangement of tungsten atoms. Single-atom defects are successfully observed for the first time during plastic deformation. Nanoribbons, which are quasi, one-dimensional structures typified by the graphene nanoribbon, have attracted an extraordinary amount of attention for their intriguing electronic properties. Other materials of interest for creating nanoribbons include layered transition-metal dichalcogenides, such as tungsten disulphide (WS 2 ), which are composed of sandwich-type basic building blocks consisting of a sheet of hexagonal close-packed transition-metal atoms between two sheets of hexagonal close-packed chalcogen atoms [1] , [2] , [3] , [4] . Such a sandwiched block is always considered to be a monolayer, although it actually consists of three sheets of atoms. There are three polytypes distinguished by different stacking sequences of the layers: trigonal symmetry, hexagonal symmetry and rhombohedral symmetry with a single layer, two layers and three layers in the unit cell, respectively. Atoms within a sheet are strongly bonded because of covalent bonds, whereas the individual sheets are stacked because of the weaker van der Waals interaction. Compared with bulk WS 2 , WS 2 nanostructures, comprising a small number of layers, could exhibit unique physical properties because of quantum confinement effects, particularly at the edges. Recently, monolayered MoS 2 and WS 2 nanoribbons encapsulated in single-walled carbon nanotubes (SWNTs) or supported on SWNTs were successfully synthesized [5] , [6] . In addition to the edges, atomic defects can also significantly affect the physical and chemical properties of such low-dimensional materials and therefore merit a thorough investigation at the atomic scale. The recent development of direct imaging and analytical techniques using a scanning transmission electron microscope (STEM) with probe-forming aberration correctors has provided direct access to information on the local atomic structure and the chemical composition at the atomic scale [7] , [8] , [9] , [10] , [11] , [12] , [13] , [14] , [15] , [16] . In particular, annular dark-field (ADF) imaging with an STEM, which was introduced by Crewe and co-workers [17] , is a powerful technique for atom-by-atom identification at a high spatial resolution. ADF was recently used to investigate the atomic structures of a boron nitride monolayer and to determine the atomic number of atoms directly on the basis of the intensity of their ADF signal [16] . Also, exit wave phase reconstruction of thin MoS 2 layers was performed using an aberration-corrected transmission electron microscopy (TEM) [18] . However, to unambiguously identify single atoms, an authentic atom-by-atom spectroscopic technique, such as electron energy-loss spectroscopy (EELS), that results in element-specific signals is required. Thus, EELS chemical analysis has been performed on nano-scale materials with atomic resolution [11] , [16] and atomic sensitivity [19] , [20] , [21] . In this study, we report successful EELS chemical mapping on an STEM to discriminate the W sites in a monolayered WS 2 nanoribbon and display an ADF-based visualization of the dynamic behaviours of single-atomic defects, allowing interpretation of the atomic process involved in slip deformation. Because of the nature of the monolayered structure, real, single-atom defects during deformation were observed successfully for the first time. Edge structures of a monolayered WS 2 nanoribbon The nanoribbons used in the experiments were confirmed to consist of WS 2 encapsulated in SWNTs after performing a preliminary experiment using TEM and energy dispersive X-ray (EDX) analysis, as shown in Supplementary Figures S1 and S2 . The cross-sectional view of the nanoribbon confirmed the monolayered structure: one sheet of W atoms sandwiched between two sheets of S atoms, which often exhibits a twisted structure ( Supplementary Fig. S2 ). 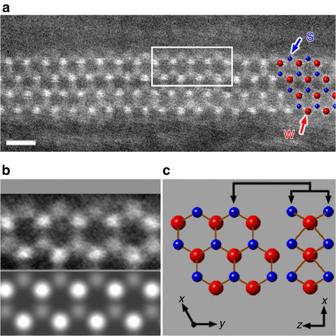Figure 1: STEM ADF image of a monolayered WS2nanoribbon encapsulated inside a SWNT. (a) The monolayered WS2nanoribbon image taken in the [001] direction. (b) An enlargement of the rectangle region shown inaand the corresponding simulated image on the lower side. (c) Model of the monolayered WS2structure (view from the [001] and [010] directions). Scale bar, 0.5 nm. The ADF image of Figure 1a illustrates the trigonal symmetry of a WS 2 nanoribbon encapsulated inside a SWNT, which confirmed the monolayered structure. The upper part of Figure 1b shows an enlarged view of the rectangular region shown in Figure 1a , and the lower part shows the corresponding simulated image. Figure 1c displays a model of the monolayered WS 2 structure with a trigonal symmetry about the [001] direction. In the ADF image, the W atoms appear brighter than the S atoms, as can be verified from the simulated image ( Fig. 1b ). The contrast of the S atoms is extremely sensitive to the nanoribbon orientation because the two S atoms cannot overlap and project at the same position if the nanoribbon is not perfectly perpendicular to the incident beam. The variable S-atom contrasts were systematically simulated in Supplementary Figure S3 . Because the S contrast in Figure 1a agrees well with the simulation, resulting in hardly any misalignment, one can reasonably conclude that all the edge atoms on the upper side consisted of S atoms (as indicated by the blue arrow). Notably, the edges of this monolayered WS 2 nanoribbon are S-terminated on one side (upper side in Fig. 1a ) and W-terminated on the other side (lower side in Fig. 1a ), and this structure does not change with the width of the monolayered WS 2 nanoribbon. It is interesting that only the zigzag edges were observed in this study. The two types of edge structures (W- and S-terminated edges) contrast with the edge structures of BN nanosheets, which also have a trigonal symmetry, but only N atoms appear at the edges [22] . This configuration of WS 2 nanoribbons, with both S and W atoms at the edges, may be the reason for their peculiar and polymorphic electronic and magnetic characteristics and therefore merits a thorough investigation. Figure 1: STEM ADF image of a monolayered WS 2 nanoribbon encapsulated inside a SWNT. ( a ) The monolayered WS 2 nanoribbon image taken in the [001] direction. ( b ) An enlargement of the rectangle region shown in a and the corresponding simulated image on the lower side. ( c ) Model of the monolayered WS 2 structure (view from the [001] and [010] directions). Scale bar, 0.5 nm. Full size image STEM–EELS analysis of a monolayered WS 2 nanoribbon Because the ADF images recorded in this study deviated from the typical high-angle annular dark-field (HAADF) condition, atoms could not be simply assigned according to the contrasts. To corroborate the ADF images, EELS chemical analysis was necessary to explicitly discriminate the elements. 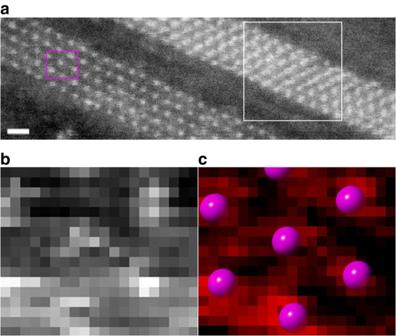Figure 2: EELS chemical map of W atoms. (a) ADF image of a monolayered WS2nanoribbon supported by a SWNT showing the spectrum image area; the referenced area marked by the white rectangle was used for drift compensation. (b) ADF image of the spectrum image area. (c) Chemical map of the WN-edge. Scale bar, 0.5 nm. Figure 2 shows a set of results from the STEM–EELS analysis of a monolayered WS 2 nanoribbon. Here, 340 EELS spectra (20×17 pixels) were recorded with a constant step of 0.03 nm in the red rectangular region from Figure 2a . Another area, marked by the white rectangle, was used for drift compensation. Figure 2b shows an ADF image that was recorded simultaneously at each pixel point, reflecting precisely the atomic positions; it can be correlated with the EELS maps. Each spectrum was subjected to a standard background stripping, and the edge intensities for the S L -edge and W N -edge were independently isolated ( Supplementary Fig. S4 ). Thus, the corresponding EELS chemical maps for these elements were constructed. Although the signal-to-noise ratios for both edges were sufficiently high to detect the presence of atoms, the chemical map does show a considerable delocalization effect. A comparison of the signal broadening in the line profiles between the ADF image and the EELS map is shown in Supplementary Figure S5 . Despite the delocalization effect, we successfully extracted the local maxima from the W N -edge map to obtain the W-atom positions ( Fig. 2c ) that perfectly coincided with the brighter contrasts in the ADF images ( Fig. 2b ). Except for the specimen/beam instabilities, the delocalization effect is the greatest obstacle in identifying the atomic position in an EELS chemical map [23] , [24] . As seen in Figure 2c , we were able to resolve the W–W distance (0.32 nm) for the W map despite the considerable delocalization effect ( Supplementary Fig. S5 ). However, the S chemical map does appear blurrier, making it rather difficult to identify the positions of the S atoms ( Supplementary Fig. S6c ). Although a lower accelerating voltage (60 kV was used) would help to reduce the delocalization of the EELS signals [21] , [25] , [26] , the delocalization effect was estimated and found to be more crucial for the S L -edge than the W N -edge. However, there might be another reason for the uncertainty of the S-atom positions in the EELS chemical map. EDX quantitative analyses clearly identified extra S atoms permeated inside the SWNTs, as shown in Supplementary Figure S7 . The extra S atoms were probably residual leftovers from the synthesis procedure and coexisted in the SWNTs, which obviously resulted in the blurry S chemical map. Figure 2: EELS chemical map of W atoms. ( a ) ADF image of a monolayered WS 2 nanoribbon supported by a SWNT showing the spectrum image area; the referenced area marked by the white rectangle was used for drift compensation. ( b ) ADF image of the spectrum image area. ( c ) Chemical map of the W N -edge. Scale bar, 0.5 nm. Full size image Various atomic defects in a monolayered WS 2 nanoribbon Atomic defects in low-dimensional materials, such as nanoribbons, can strongly affect the physical properties, such as mechanical or transport properties, and chemical properties much more than those in bulk materials. Therefore, an investigation into the nature of atomic defects at the atomic scale is essential. Various point defects can be induced in low-dimensional material when the beam current is intentionally increased. In this study, we recorded the dynamic behaviours of the atomic defects that were in continuous motion during the observation. 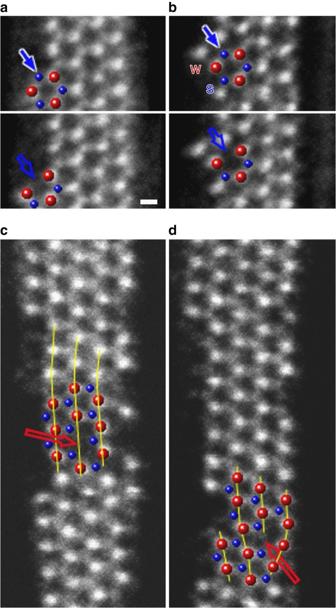Figure 3: Single atomic defect in a monolayered WS2nanoribbon. (a,b) Dynamic process of the atomic defects created at S sites. (a) Edge-atom loss of S and (b) vacancy creation. (c) Simple W monovacancy and (d) W vacancy with a large distortion in the surrounding lattice. The open blue arrows indicate the loss of S atoms and the red open arrows indicate W vacancies. Scale bar, 0.2 nm. Figure 3 shows the atomic process of vacancy creation in a monolayered WS 2 nanoribbon. Figures 3a,b show two different processes involved in knocking out S atoms. Figure 3a shows the states before and after the loss of an S atom at an edge, which occurred within 1 s (the typical time interval for one ADF image scan). A monovacancy of an S atom was also created, as shown in Figure 3b , in which the S atom and the S vacancy are indicated by the solid and empty arrows, respectively. Note that the S-vacancy creation does not induce a large distortion in the WS 2 nanoribbon. Figure 3: Single atomic defect in a monolayered WS 2 nanoribbon. ( a , b ) Dynamic process of the atomic defects created at S sites. ( a ) Edge-atom loss of S and ( b ) vacancy creation. ( c ) Simple W monovacancy and ( d ) W vacancy with a large distortion in the surrounding lattice. The open blue arrows indicate the loss of S atoms and the red open arrows indicate W vacancies. Scale bar, 0.2 nm. Full size image In contrast, the creation of a W vacancy induces a drastic structural deformation in the nanoribbons. Nanoribbons containing two different W vacancies are shown in Figures 3c,d (marked by red arrows). Note that the vacancies were recorded in different regions on the same ribbon. The W vacancy in Figure 3c is a simple monovacancy; that is, all the lattice points remained unchanged except for the missing W atom. However, one can notice considerable elastic deformation of the nanoribbon, seen as a small bend in the middle. The other W vacancy, shown in Figure 3d , is more interesting because it induced a large structural deformation. In the W vacancy region (indicated by the open arrow), the atomic rows became mismatched, and a 'dislocation' was induced, as shown by the yellow lines. Therefore, all the lattice points surrounding the W vacancy became relaxed to accommodate the 'dislocation' core. We call this a dislocation because in the projection direction, it is similar to a dislocation in ordinary three-dimensional crystals. However, it should be noted that the dislocation here indicates a point defect. An S vacancy may also be associated with this dislocation to create a more relaxed structure because one of the S lattice points seems to have disappeared. Another interesting phenomenon concerning the atomic defects in motion is the migration of edge atoms. 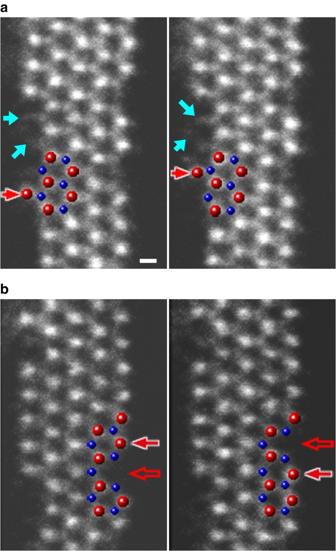Figure 4: Two sequential ADF images for the edge-atom migration. (a) Migration of a W atom along the S-terminated edge. (b) Migration of a W atom/vacancy along the W-terminated edge. The cyan arrows indicate single S atoms. Scale bar, 0.2 nm. Two sets of ADF images showing the migration of a W atom and/or vacancy are shown in Figure 4 . This W-atom migration exhibited different behaviour depending on whether the edge was W-terminated or S-terminated. Figure 4a shows an extra W-atom migrating on an S-terminated edge. In the two sequential ADF images recorded at a 1-s interval, a W atom instantly jumped from an edge position to the next site (indicated by red arrows). This W atom was almost bare, in which only a single neighbouring S site (likely two S atoms) was available to bond. The second example shows a W atom jumping to an adjacent vacancy along a W-terminated edge and leaving behind another vacancy—as if the W atom and vacancy exchanged positions (solid and open arrows in Fig. 4b ). In this case, the W atom had at least two neighbouring S sites and would have required greater energy to migrate than in the previous case. Figure 4: Two sequential ADF images for the edge-atom migration. ( a ) Migration of a W atom along the S-terminated edge. ( b ) Migration of a W atom/vacancy along the W-terminated edge. The cyan arrows indicate single S atoms. Scale bar, 0.2 nm. Full size image Finally, we investigated the atomic process involved in slip deformation, which was frequently observed during the STEM observations of the nanoribbons. Generally, slip deformation occurs in crystals that are subject to a tensile stress larger than the critical shear stress. Although most types of plastic deformations in crystalline materials are believed to originate from the sliding of dislocations, the atomic processes involved have never been directly observed thus far. 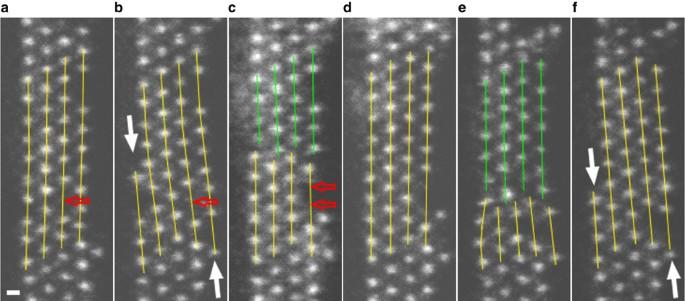Figure 5: A sequential set of ADF images depicting the atomic process during slip deformation. (a) W vacancy created (0 s). (b) Slip deformation (1 s) with an edge-atom migration. (c) Vacancy migration and emergence of the slip-line (or the lattice mismatch; 11 s). (d) Dynamic recovery (12 s) and the mismatch disappears. (e) Another slip-line appears (25 s) and then (f) the slip deformation process ended (26 s). Scale bar, 0.2 nm. The six sequential ADF images in Figure 5 show a nanoribbon exhibiting slip deformation. Only the W atoms can be seen because the S-atom positions could not be properly identified given the short scanning time (1 s per frame, whereas the scanning time was 6 s per frame in Fig. 3 and 1.5 s per frame in Fig. 4 ) and the possible deflection from the [001] direction. In Figure 5a , a W vacancy (indicated by an open arrow) and an extra W atom at the edge appeared in the nanoribbon, with four atomic rows of W (indicated by the yellow lines). A relaxation suddenly occurred around the vacancy, together with a reorganization of the atomic rows ( Fig. 5b ). Then, the W vacancy was pushed to the edge (indicated by the open arrows in Fig. 5c ) and a 'partial slip,' indicated by the green and yellow lines, appeared at the same time. The dynamic recovery of the atomic rows may occur instantly due to the slip back of the lattice mismatch ( Fig. 5d ). Another partial slip emerged just after the recovery ( Fig. 5e ), and the slip deformation was complete when extra atomic rows appeared, indicated by white arrows ( Fig. 5f ). Figure 5: A sequential set of ADF images depicting the atomic process during slip deformation. ( a ) W vacancy created (0 s). ( b ) Slip deformation (1 s) with an edge-atom migration. ( c ) Vacancy migration and emergence of the slip-line (or the lattice mismatch; 11 s). ( d ) Dynamic recovery (12 s) and the mismatch disappears. ( e ) Another slip-line appears (25 s) and then ( f ) the slip deformation process ended (26 s). Scale bar, 0.2 nm. Full size image Notably, there were additional atom-like features showing weak contrasts at the edge of the WS 2 ribbon, as shown in Figures 3c,d and 4a and indicated by the cyan arrows. Such contrasts were weaker than those of the two S atoms. According to the EDX analyses, there were no other elements inside the SWNT except for C, O, S and W. Contrast intensity ratios of the unknown atoms to the double S atoms were measured from the experimental ADF images and compared with the contrast ratios of a single S atom to double S atoms (S(1)/S(2)), single oxygen atom to double S atoms (O/S(2)) and single carbon atom to double S atoms (C/S(2)) calculated from the simulated ADF image, as shown in Supplementary Figure S8 . The contrast ratio of the unknown atoms to the double S atoms fits well with that of the S(1)/S(2) from the calculation. Therefore, we can reasonably conclude that these atom-like features with a weaker contrast are due to single S atoms. The slip deformation investigated here does not represent a normal deformation process caused by an external shear force, but was indeed generated by the dynamic movements of the atomic defects due to the incident electron beam. Such an electron beam-induced deformation has also been observed in a bi-crystal of gold [27] . Nevertheless, this observation provides deeper insights into the behaviour of active atomic defects during deformation processes and could eventually explain how they can induce macroscopic deformation. The low-accelerating voltage used here (60 kV) was beneficial because it reduced the probability of a point defect being induced by knock-on damage, making such an in situ observation at the atomic level possible. We anticipate that further decreasing the accelerating voltage will also be advantageous in reducing the EELS delocalization effect, which is currently a major obstacle to single-atomic elemental analysis. If this obstacle can be overcome, dynamic analysis of active point defects may become more common. Synthesis and characterization SWNTs produced by the arc-discharge method were used as templates for the fabrication of the WS 2 nanoribbons. Typically, 5 mg of carbon nanotubes (CNTs) were added to 10 ml of a saturated, aqueous solution of H 3 PW 12 O 40 . Then, the solution was sonicated for 1 h and refluxed for 2 h. The WS 2 nanoribbons were produced by heating the CNTs filled with H 3 PW 12 O 40 at 800 °C in a H 2 S/H 2 atmosphere for 2 h. STEM and EELS observations A JEOL 2100F (JEOL) with a cold field-emission gun equipped with a newly designed aberration corrector (the DELTA-corrector) was operated at 60 kV. Typically, a 0.11-nm resolution was achieved for the STEM ADF imaging. A Gatan GIF Quantum (Gatan) was used for the EELS chemical analyses. The inner and outer collection angles for the ADF image (β 1 and β 2 ) were 45 mrad and 100 mrad, respectively. The beam current was 10 pA for the ADF imaging and 20 pA for the EELS chemical analysis. How to cite this article: Liu, Z. et al . Identification of active atomic defects in a monolayered tungsten disulphide nanoribbon. Nat. Commun. 2:213 doi: 10.1038/ncomms1224 (2011).